Single-atomic-site platinum steers photogenerated charge carrier lifetime of hematite nanoflakes for photoelectrochemical water splitting Although much effort has been devoted to improving photoelectrochemical water splitting of hematite (α-Fe 2 O 3 ) due to its high theoretical solar-to-hydrogen conversion efficiency of 15.5%, the low applied bias photon-to-current efficiency remains a huge challenge for practical applications. Herein, we introduce single platinum atom sites coordination with oxygen atom (Pt-O/Pt-O-Fe) sites into single crystalline α-Fe 2 O 3 nanoflakes photoanodes (SAs Pt:Fe 2 O 3 -Ov). The single-atom Pt doping of α-Fe 2 O 3 can induce few electron trapping sites, enhance carrier separation capability, and boost charge transfer lifetime in the bulk structure as well as improve charge carrier injection efficiency at the semiconductor/electrolyte interface. Further introduction of surface oxygen vacancies can suppress charge carrier recombination and promote surface reaction kinetics, especially at low potential. Accordingly, the optimum SAs Pt:Fe 2 O 3 -Ov photoanode exhibits the photoelectrochemical performance of 3.65 and 5.30 mA cm −2 at 1.23 and 1.5 V RHE , respectively, with an applied bias photon-to-current efficiency of 0.68% for the hematite-based photoanodes. This study opens an avenue for designing highly efficient atomic-level engineering on single crystalline semiconductors for feasible photoelectrochemical applications. Photoelectrochemical (PEC) water splitting has attracted great promises in recent years for sustainable hydrogen production [1] , [2] , [3] , [4] , [5] , in which the fabrication of the suitable semiconductor photoanodes with sufficient light absorption and efficient charge carrier transport is becoming increasingly important for achieving high solar-to-hydrogen (STH) conversion efficiency [6] , [7] , [8] , [9] , [10] . Many metal oxide semiconductors such as TiO 2 [11] , [12] , [13] , α-Fe 2 O 3 [14] , [15] , [16] , BiVO 4 [17] , [18] , [19] , and WO 3 [20] , [21] , [22] , have been considered as promising candidates owing to their availability, facile preparation, and oxidative stability. Especially, hematite (α-Fe 2 O 3 ), a n-type semiconductor with a small band gap of ~2.1 eV, can absorb a large portion of the solar spectrum and allow a theoretical STH efficiency of 15.5% under standard sunlight illumination [23] , [24] , [25] , [26] . However, its short hole diffusion length, poor charge carrier conductivity, and sluggish oxygen evolution reaction kinetics limit the photocurrent of α-Fe 2 O 3 far below its theoretical value of 12.4 mA cm −2 [27] , [28] . Especially, the low electron mobility (~10 −2 cm 2 V −1 s −1 ) as one of the main intrinsic drawbacks significantly impedes its PEC performance [29] , [30] , [31] . To enhance the electron mobility of photoelectrode, doping elements (e.g., Ti [32] , [33] , [34] , Sn [35] , [36] , [37] , Zr [38] , La [39] , Ta [27] , [40] , B [41] , and P [31] ) have been adapted to substantially ameliorate the photo-efficiency of α-Fe 2 O 3 . For example, nonmetallic P doping has a superior activity owing to the strong covalent interaction between P and O, which boosted fast electron carriers and avoided the formation of deep electron trapping sites in α-Fe 2 O 3 [31] . Although these doping elements can improve more or less the electrical conductivity and charge transfer of α-Fe 2 O 3 , all the dopants in the photoelectrodes reported so far are clusters or bigger than clusters. As a result, not only the improvement of PEC is limited, but also the band bending caused by these clusters decreases the width of space-charge layer which limits the number of the carriers inside of the layer. In addition, these traditional dopants have not much influence on onset potential (generally located at 0.8–1.0 V RHE ). The onset potential further influences the applied bias photon-to-current efficiency (ABPE) of α-Fe 2 O 3 due to the surface and bulk trap states [3] , [42] , the high onset potential causing to the low ABPE. Therefore, additional strategies are desirable to improve the charge transfer efficiency and ABPE value. Recently, engineering single atom catalysts have been widely used to enhance the oxygen evolution reaction performances. Unsaturated coordination environments of single atoms often function as active sites, influencing the catalytic performances [43] , [44] . However, most single atoms are incorporated into amorphous catalyst layers, and no reports are related to single atom doping semiconductors. For example, atomically dispersed Ni-N 4 sites coordinated with oxygen atom have promoted photogenerated charge separation and thus improved PEC performance of BiVO 4 [45] . The single atom catalysts grown on an amorphous support act as the charge transfer layer, and the construction of single-atomic Ni-N 4 -O moiety is located at the interface of photoelectrode/oxygen evolution cocatalyst (OEC). In fact, more serious recombination usually happens in the bulk materials. To this end, it is highly desirable to design single metal atoms doped into photoelectrode to efficiently transfer carrier from the bulks to the photoelectrode/electrolyte interfaces, and improve the OER and PEC performances. Herein, we develop a versatile strategy to engineer single platinum atom sites coordinated with an oxygen atom (Pt-O) incorporated into single crystalline hematite photoanodes by using 2,2-bipyridine as the ligand to chelate Pt cations, followed by the inert atmosphere treatment to remove the ligand. The construction of single atomic Pt-O coordination in Fe 2 O 3 nanoflakes (SAs Pt:Fe 2 O 3 ) owns few deep electron trapping sites in hematite. 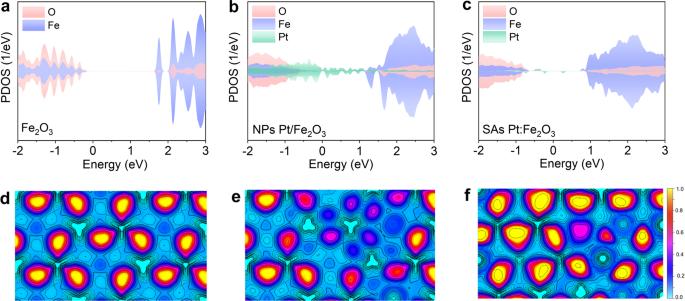Fig. 1: Electronic structures of Fe2O3, NPs Pt/Fe2O3, and SAs Pt:Fe2O3. a–cProjected density of states (PDOS) states ofaFe2O3,bNPs Pt/Fe2O3, andcSAs Pt:Fe2O3,d–felectron density distribution plots ofdFe2O3,eNPs Pt/Fe2O3, andfSAs Pt:Fe2O3. Accordingly, the SAs Pt:Fe 2 O 3 with the surface oxygen vacancies can achieve the photocurrent density of 3.65 mA cm −2 at 1.23 V RHE with a ABPE of 0.68%, which is more than double most of the previously reported values of the doped Fe 2 O 3 -based photoanodes (Supplementary Table 1 ), and even superior to the cocatalysts decorated Fe 2 O 3 -based photoanodes. X-ray absorption fine structure analysis, time-resolved spectroscopic investigation, and time domain density functional theory and nonadiabatic molecular dynamics calculations have demonstrated that the improved PEC activity can be ascribed to the construction of the single-atomic Pt-O and Pt-O-Fe in Fe 2 O 3 , which facilitates the hole transfer from Fe 2 O 3 bulk to interface, extends the charge carrier lifetime, and accelerates the reaction kinetics for PEC water splitting. Electronic structure of Fe 2 O 3 and Pt doped Fe 2 O 3 Using the density functional theory (DFT) method, we firstly calculated the projected density of states (PDOS) and electron localization function (ELF) to determine if the loading of Pt nanoparticles (NPs) and single atoms (SAs) can influence the electronic structure and electron mobility of Fe 2 O 3 geometries, and the samples are labeled as NPs Pt/Fe 2 O 3 and SAs Pt:Fe 2 O 3 (Supplementary Fig. 1a–c ). The computed direct band gap of Fe 2 O 3 is approximately 2.0 eV (Fig. 1a ), agreeing with the value reported in the literature (2.1 eV) [14] , [15] . For the NPs Pt/Fe 2 O 3 , partial Pt atoms are bonded to surface oxygens, whilst others exhibit metallic properties, forming the Pt-Pt bonds. The Pt NPs introduce almost continuous states between the band gap of Fe 2 O 3 (Fig. 1b ), promoting the photogenerated electrons transferring from Fe 2 O 3 to Pt NPs. However, the state created by Pt NPs can act as the charge recombination center. Further downsizing the Pt nanoparticles to single atomic level, Pt atoms form Pt-O covalent bonds with O atoms, which create several charge trapping states within the bandgap compared to that of NPs Pt/Fe 2 O 3 (Fig. 1c ). These trapping states primarily composed of SAs Pt atoms, can trap the photogenerated charge carriers and accelerate the electron-hole separation (discussion in the following). Moreover, ELF shows that doping Pt reduces the electron localization in regard to that of the pristine Fe 2 O 3 (Fig. 1d–f ), benefiting to improve electron transport rate. Comparatively, the strong Pt-O and metal-metal interaction exist in NPs Pt/Fe 2 O 3 (Fig. 1e ), while the latter vanishes in SAs Pt:Fe 2 O 3 (Fig. 1f ). These results confirm that single atomic Pt doping can facilitate the electron separation and transfer in contrast to traditional doping engineering in term of improving performance. Fig. 1: Electronic structures of Fe 2 O 3 , NPs Pt/Fe 2 O 3 , and SAs Pt:Fe 2 O 3 . a – c Projected density of states (PDOS) states of a Fe 2 O 3 , b NPs Pt/Fe 2 O 3 , and c SAs Pt:Fe 2 O 3 , d – f electron density distribution plots of d Fe 2 O 3 , e NPs Pt/Fe 2 O 3 , and f SAs Pt:Fe 2 O 3 . Full size image Synthesis and characterization of SAs Pt:Fe 2 O 3 Motivated by the theoretical calculations, SAs Pt:Fe 2 O 3 photoanode was synthesized as illustrated in Fig. 2a . To begin with, one-dimensional single-crystalline Fe 2 O 3 nanoflakes were formed by a thermal treatment at 400 °C for 3 h in air (Supplementary Fig. 2 ), and subsequently were immersed in the solution of 2,2-bipyridine as the ligand to chelate Pt cations. The ligand was removed under Ar atmosphere at 330 °C to obtain isolated single-atomic Pt doped Fe 2 O 3 (Supplementary Fig. 3 ). The NPs Pt/Fe 2 O 3 was prepared as the thermal temperature was 400 °C (Supplementary Fig. 4 ). X-ray diffraction (XRD) pattern of SAs Pt:Fe 2 O 3 displays the Fe 2 O 3 (JCPDS No. 33-0664), Fe 3 O 4 (JCPDS No. 19-0629), and Fe peaks (Supplementary Fig. 4d ). The formation of Fe 3 O 4 originated from the thermal annealing treatment owing to the oxygen diffusion from the surface to the bulk material. Fe 3 O 4 is not photoactive for photoelectrochemical performance, while it can be assured that it is more conducive than the Fe 2 O 3 , and acts as a conductive layer to transfer charge carrier from the Fe 2 O 3 to the back side [46] . Scanning electron microscopy (SEM) images exhibit one dimensional nanoflakes structure with a length of 1.5–2.5 μm on SAs Pt:Fe 2 O 3 (Fig. 2b and Supplementary Fig. 5 ). The aberration-corrected high-angle annular dark-field scanning transmission electron microscopy (AC-HAADF-STEM) images reveal a high degree of single atom dispersion for SAs Pt:Fe 2 O 3 (Fig. 2c–e and Supplementary Fig. 6 ), where the Pt atoms are uniformly dispersed at the Fe atom positions (Fig. 2f, g ). One can see that the edge of nanoflakes presents the defected structure decorated with the isolated Pt atoms (Fig. 2d and Supplementary Fig. 7 ). Element mapping shows the homogeneous distribution of Fe, O, and Pt species across the whole nanoflakes (Fig. 2h ), indicative of the presence of single atom (Supplementary Fig. 8 ). Induced coupled plasma-mass spectrometry analysis shows ~4 at.% of Pt content on SAs Pt:Fe 2 O 3 . On the contrary, significant aggregation of Pt species with a size of 5–10 nm can be observed on NPs Pt/Fe 2 O 3 (Supplementary Figs. 9 – 11 ). The controllable experiment using the same manner without 2,2-bipyridine results in the formation of Pt nanoparticles (Supplementary Fig. 12 ). It should be noted that the use of 2,2-bipyridine and low annealing treatment are the critical factors to realize the single atom sites and maintain the dispersion of Pt species. This is a feasible approach of tailoring Pt single atoms doping into single crystalline photoelectrodes. Fig. 2: Characterization of SAs Pt:Fe 2 O 3 . a Schematic illustration for the synthesis of SAs Pt:Fe 2 O 3 . Color codes: grey (Pt), green (Cl), blue (N), and purple (C); b SEM images; c – e high resolution HAADF STEM images. A large numbers of Pt atoms were atomically dispersed on the Fe 2 O 3 as observed in c . Inset of e shows the FFT pattern; f , g the lines represent the line profiles from HAADF intensity analysis labeled in e ; h elemental mapping. Scale bars in b – e , and h are 200 nm, 5 nm, 500 pm, 500 pm, and 20 nm, respectively. Full size image X-ray photoelectron spectra (XPS) and X-ray absorption fine structure (XAS) spectroscopy were used to probe the local coordination chemistry of the Pt species. The binding energies of Pt 4f 7/2 (72.80) and Pt 4f 5/2 peaks (76.10 eV) on SAs Pt:Fe 2 O 3 are higher than those of metallic Pt 0 and lower than those of Pt 4+ (Fig. 3a ), indicating the presence of SAs Pt in hematite. The only Pt 4f peaks representing the metallic Pt appear in NPs:Fe 2 O 3 (Supplementary Fig. 13 ). To further provide the evidence of single atom, Fig. 3b exhibits two peaks at 1.94 Å and 2.84 Å in the Pt L -edge X-ray absorption fine structure (EXAFS) spectrum of SAs Pt:Fe 2 O 3 . The first shell originates from the coordination of Pt atom to oxygen (Pt-O), and the second shell fits for the Pt-O-Fe with a comparison between Pt-O-Fe and Pt-Pt coordination models, consistent with the analysis of the dispersed Pt atoms from HADDF-STEM images (Fig. 2c ). The contribution of Pt-O and Pt-O-Fe comes from the interaction between single Pt site and oxygen/iron atoms on Fe 2 O 3 . The normalized X-ray absorption near-edge structure (XANES) spectra exhibit the intensity of SAs Pt:Fe 2 O 3 located at Pt foil and PtO 2 (Fig. 3c ), manifesting that the valence of Pt is lower than +4. The R space fitting and EXAFS fitting results suggest that the calculated structure is Pt-O and Pt-O-Fe (Supplementary Fig. 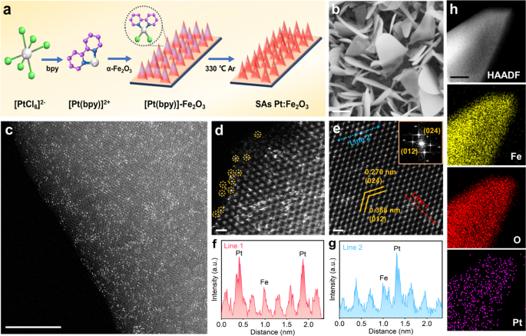Fig. 2: Characterization of SAs Pt:Fe2O3. aSchematic illustration for the synthesis of SAs Pt:Fe2O3. Color codes: grey (Pt), green (Cl), blue (N), and purple (C);bSEM images;c–ehigh resolution HAADF STEM images. A large numbers of Pt atoms were atomically dispersed on the Fe2O3as observed inc. Inset ofeshows the FFT pattern;f,gthe lines represent the line profiles from HAADF intensity analysis labeled ine;helemental mapping. Scale bars inb–e, andhare 200 nm, 5 nm, 500 pm, 500 pm, and 20 nm, respectively. 14 and Supplementary Table 2 ). SAs Pt:Fe 2 O 3 exhibits Pt-O bonding with coordination number (CN) approaching 4.5 at 1.94 Å, and Pt-O-Fe bonding with CN approaching 1.0 at 2.84 Å in second coordination shell, clearly demonstrating the formation of single atom on hematite. Owing to the powerful resolution in both k and R spaces, the Pt L edge wavelet transform extended EXAFS (WT-EXAFS) was employed to investigate the atomic configuration of SAs Pt:Fe 2 O 3 with the references of Pt foil and PtO (Fig. 3d–f ). For the Pt L edge wavelet transform of χ ( k ) spectra of SAs Pt:Fe 2 O 3 , one highest merged scattering path signal of Pt-O bond located at [ χ ( k ), χ ( R )] of [6.0, 2.02] is observed, and a low scattering path signal of Pt-O-Fe bond located at [ χ ( k ), χ ( R )] of [6.0, 3.0] can be seen (Fig. 3f ). The characteristic scattering path signal of Pt-Pt bond in the Pt foil is located at [7.4, 2.80] (Fig. 3d ), and it is not detected on SAs Pt:Fe 2 O 3 . The characteristic scattering path signal of Pt-O bonds in the PtO is located at [6.0, 2.0] (Fig. 3e ). The WT-EXAFS analysis determines the radial distance and k space resolution, confirming the coexistence of Pt-O and Pt-O-Fe without Pt-Pt in SAs Pt:Fe 2 O 3 . The above analyses demonstrate that the dispersed Pt atoms are in the form of Pt-O and Pt-O-Fe bonds in the hematite nanoflakes. Fig. 3: Coordination environment analysis of SAs Pt:Fe 2 O 3 . a Pt 4f XPS spectra; b Fourier-transformed R -space of the experimental Pt K -edge EXAFS signals; c normalized XANES spectra; d – f 3D contour WT-EXAFS maps with 2D projection of d Pt foil, e PtO, and f SAs Pt:Fe 2 O 3 . g free energies of OER reaction steps occurring on Pt-O or Pt-O-Fe active sites in SAs Pt:Fe 2 O 3 . Full size image To investigate the real reaction path of four-electron oxygen evolution reaction (OER) in SAs Pt:Fe 2 O 3 , we calculated the thermodynamic free energy diagrams for OER. The side view structures of *OH, *O, and *OOH absorbed on SAs Pt:Fe 2 O 3 surface are shown in the inset of Fig. 3g . The calculated data in Fig. 3g demonstrate that there are two OER paths (first OER path: Pt-OH → PtOFe → PtOOH → O 2 ; second OER path: Pt-OH → PtO → PtOOH → O 2 ) in SAs Pt:Fe 2 O 3 surface. Typically, the higher energy barrier of rate-determining steps, the larger overpotentials ( η ) for OER. As seen in Fig. 3g , we can conclude that the energy barrier of *O intermediate formation in the first OER path (2.07 eV) is lower than that of *OOH intermediate formation in the second OER path (2.48 eV). Thus, the η of first OER path (0.84 V) is lower than that of second OER path (1.25 V). The distinct 0.41 V drop in η shows that the first OER path is the real reaction path in SAs Pt:Fe 2 O 3 , indicating that Pt-O-Fe is the crucial active site which can promote the surface OER kinetics and improve the solar water splitting activity. Photoelectrochemical performance The PEC performances were investigated in a three-electrode cell (Supplementary Fig. 15 ). Figure 4a shows the photocurrent-potential ( J-V ) curves of the photoanodes in 1 M KOH under AM 1.5G (100 mW cm −2 ) simulated sunlight. 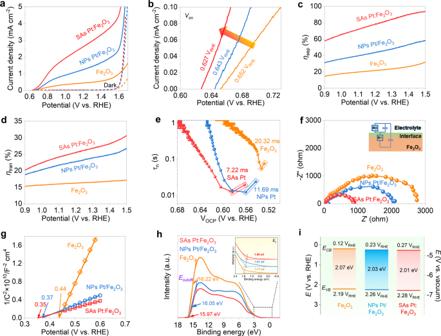Fig. 4: PEC performances and band edge energetics of Fe2O3, NPs Pt/Fe2O3, and SAs Pt:Fe2O3. aJ-Vcurves;bextractedVon;ccharge separation efficiencies;dcharge transfer efficiencies;eOCP-derived carrier transfer lifetimes;fPEIS at 1.23 VRHE. Inset shows the circuit;gMott-Schottky plots;hUPS spectra. The black dashed lines indicate the area shown in zoomed-in image in the inset ofh;iband diagrams determined from UV-vis absorption and UPS measurements. All electrochemical measurements were performed in 1 M KOH under AM 1.5G illumination (100 mW cm−2). The pristine Fe 2 O 3 displays a photocurrent density of 0.45 mA cm −2 at 1.23 V RHE with an onset potential ( V on ) of 0.652 V RHE . With the introduction of Pt dopant into hematite, both NPs and SAs enhance the photocurrent densities of hematite, accompanied by the negative shift of V on , indicating the fast charge transfer by Pt incorporation. Dark current densities for both samples are also remarkably improved with a cathodic shift of approximately 58 mV at 0.5 mA cm −2 (Supplementary Fig. 16 ). The optimum SAs Pt:Fe 2 O 3 shows a photocurrent density of 2.71 mA cm −2 at 1.23 V RHE (Supplementary Fig. 17 ), higher than that of NPs Pt/Fe 2 O 3 (1.29 mA cm −2 ). Moreover, the V on of SAs Pt:Fe 2 O 3 (0.627 V RHE ) is found to be negatively shifted by 25 and 16 mV relative to those of the pristine Fe 2 O 3 and NPs Pt/Fe 2 O 3 (Fig. 4b ), suggesting the enhanced surface water oxidation kinetics, especially the surface edge with the substitution of single atomic Pt (Fig. 2d ). The improved photocurrent and the reduced V on increase ABPE with a maximum value of 0.51% (Supplementary Fig. 18 ), which surpasses the previously reported the highest value of 0.31% [27] . Besides, the current spike on SAs Pt:Fe 2 O 3 ( i / i 0 = 0.91) is reduced from the chopped J-V plots (Supplementary Fig. 19 ), indicating promoting sluggish water oxidation by single atomic Pt. Fig. 4: PEC performances and band edge energetics of Fe 2 O 3 , NPs Pt/Fe 2 O 3 , and SAs Pt:Fe 2 O 3 . a J-V curves; b extracted V on ; c charge separation efficiencies; d charge transfer efficiencies; e OCP-derived carrier transfer lifetimes; f PEIS at 1.23 V RHE . Inset shows the circuit; g Mott-Schottky plots; h UPS spectra. The black dashed lines indicate the area shown in zoomed-in image in the inset of h ; i band diagrams determined from UV-vis absorption and UPS measurements. All electrochemical measurements were performed in 1 M KOH under AM 1.5G illumination (100 mW cm −2 ). Full size image To understand the charge character by the influence of SAs Pt, charge separation efficiency ( ƞ sep ) and charge transfer efficiency ( ƞ tran ) were calculated, and derived from the J-V curves measured in a hole scavenger-containing electrolyte (Supplementary Fig. 20 ). The ƞ sep points to the hole extraction from the excited Fe 2 O 3 to the surface. From Fig. 4c , Pt doping dramatically improves the ƞ sep in the entire voltage region. SAs Pt:Fe 2 O 3 presents higher ƞ sep values in relative to the traditional particles doping, reaching to 80.1% at 1.23 V RHE , while NPs Pt/Fe 2 O 3 arrives to 44.1% of the same potential. Single atom edging at the surface also plays a vital role for the hole trapping to the surface for water oxidation. Besides, SAs Pt:Fe 2 O 3 exhibits a ƞ tran value of 25.8% at 1.23 V RHE (Fig. 4d ), higher than that of NPs Pt/Fe 2 O 3 (23.0%), indicating that the fraction of holes reaches to the semiconductor/electrolyte interface without significant recombination in the bulk material. All these results confirm that adjusting the coordination environment via atom-level regulation for PEC water splitting evidently promotes to the charge separation/transfer and realizes efficient energy conversion. Open circuit potential (OCP) transient decay profile provides an additional information on the photogenerated charge carrier behavior. The OCP in dark is positive and then shifts to the negative direction under illumination (Supplementary Fig. 21a ), which is caused by built-in electric field generated by the photo-generated carriers [27] . SAs Pt:Fe 2 O 3 presents a strikingly accelerated OCP decay as terminating the illumination in relative to NPs Pt/Fe 2 O 3 , representing a large photovoltage generation ( Δ OCP = OCP dark - OCP light ). Charge transfer and recombination are principally two competing processes that determine the water oxidation rate on the photoanode surface. To further clarify the charge recombination rate at the semiconductor/electrolyte junction, the carrier transfer lifetime was calculated from the derived-OCP values, as depicted in Fig. 4e (see details for supporting information). NPs Pt/Fe 2 O 3 displays a carrier lifetime of 11.69 ms when illumination was removed, one time lower than the pristine Fe 2 O 3 (20.32 ms). SAs Pt substitution continues to reduce upon 7.22 ms on Fe 2 O 3 , indicating effective charge separation and fast transfer kinetics. In addition, the incident photon-to-current conversion efficiency (IPCE) on SAs Pt:Fe 2 O 3 is remarkably improved over the entire range of 340-600 nm (Supplementary Fig. 21b ). Figure 4f shows the photoelectrochemical impedance spectroscopy (PEIS) for the corresponding photoanodes, and the equivalent circuit was employed to fit the Nyquist plots of PEIS (inset of Fig. 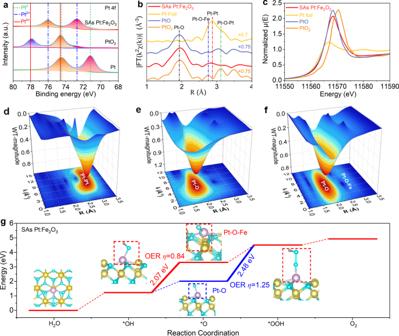4f ). Fig. 3: Coordination environment analysis of SAs Pt:Fe2O3. aPt4fXPS spectra;bFourier-transformedR-space of the experimental PtK-edge EXAFS signals;cnormalized XANES spectra;d–f3D contour WT-EXAFS maps with 2D projection ofdPt foil,ePtO, andfSAs Pt:Fe2O3.gfree energies of OER reaction steps occurring on Pt-O or Pt-O-Fe active sites in SAs Pt:Fe2O3. SAs Pt:Fe 2 O 3 exhibits a considerably lower resistance (546.50 Ω) than NPs Pt/Fe 2 O 3 (809.80 Ω) and Fe 2 O 3 (2719.40 Ω), as summarized in Supplementary Table 3 . And, SAs Pt:Fe 2 O 3 remains a relatively stable photocurrent for 10 h durability (Supplementary Fig. 22a ). The gases produced from the working and counter electrodes present the evolved O 2 and H 2 with a ratio of 2:1 with the Faraday efficiencies of gas productions closed to 100% (Supplementary Fig. 22b ). In fact, anion and cations species modulation allow to induce extra electrons near Fe 3+ sites to form Fe 2+ sites, which can enhance the electrical conductivity of Fe 2 O 3 . However, high amount metal doping would principally induce the recombination centers by creating inter-bandgap energy states since the Fe 2+ sites are near to the surface region, causing trapping states and high overpotential for water oxidation. The coordination of single atomic-level Pt substitution for Fe 3+ can avoid the high concentration of doping to a certain degree, which increases the polaron hopping probability, and feasibly enhances the photogenerated charge carrier rate for PEC reaction, consistent with the DFT calculation. On the other hand, atom-level substitution near to the surface would inhibit the interfacial charge recombination, which is reflected by the low V on . The flat band potentials ( E fb ) of SAs Pt:Fe 2 O 3 and NPs Pt/Fe 2 O 3 were conducted by Mott-Schottky measurement. E fb is cathodically shifted since Pt was induced (Fig. 4g ), coincided with the shift of V on from the J-V plot (Fig. 4b ). SAs Pt:Fe 2 O 3 has shown a lower E fb (0.35 V RHE ) than NPs Pt/Fe 2 O 3 (0.37 V RHE ), manifesting the change in the band energetics. Besides, the similar slopes of Mott–Schottky plots represent the resembled carrier concentration, implying the close donor densities in the supporting materials loading with Pt nanoparticles and single-atom. Ultraviolet photoelectron spectroscopy (UPS) and ultraviolet-visible (UV-Vis) absorption were implemented to illustrate the band edge positions of the photoanodes. Tauc plots of photoanodes declare the band gaps of the pristine Fe 2 O 3 , NPs Pt/Fe 2 O 3 , and SAs Pt:Fe 2 O 3 are 2.07, 2.03, and 2.01 eV (Supplementary Fig. 23 ), respectively, coherent with the decreased slopes of Mott-Schottky (Fig. 4g ). The work functions of the samples were determined by subtracting the cutoff energies ( E cutoff ) from the UPS curves (Fig. 4h ). The positions of the valence band maxima in regard to the Fermi levels were derived from the onset of valence band photoemission on the low binding energy edges of UPS spectra (inset of Fig. 4h ). Based on these results, the determined band positions for the corresponding samples are summarized in Fig. 4i and Supplementary Table 4 , according to the literatures reported [3] , [47] . One can see that tailoring Pt-O sites can influence the band structure, promote the charge separation, and accelerate the photogenerated holes transferring to the semiconductor/electrolyte surface for water oxidation, therefore enhancing PEC performance. IMPS and TAS analysis for carrier kinetics Furthermore, we performed intensity modulated photocurrent spectroscopy (IMPS) and transient absorption spectroscopy (TAS) to understand the charge carrier kinetics in various Fe 2 O 3 photoanodes. The semicircle coincides with the competition between interfacial carrier transfer and electron-hole recombination (Supplementary Fig. 24 ). The frequency of the maximum imaginary is associated with the sum of charge transfer ( k trans ) and recombination ( k rec ) rate constants ( k trans + k rec ) [48] , [49] , [50] . The ratio of k trans /( k trans + k rec ) is taken by comparing the instantaneous photocurrent and steady-state photocurrent. SAs Pt:Fe 2 O 3 exhibits the highest k trans values over the measured potential range (Fig. 5a ), indicating that single atoms speed up the charge carrier mobility and quickly transfer from the bulk material to the surface or to the back contact. By contrast, the k rec of SAs Pt:Fe 2 O 3 is lower than that of NPs Pt/Fe 2 O 3 , and almost overlapped with that of the pristine Fe 2 O 3 in the potential of 0.8–1.1 V RHE (Fig. 5b ), indicating high charge transfer rate of SAs Pt:Fe 2 O 3 . Further considering surface substitution by SAs Pt, Fermi level pinning effect caused by surface states can be eliminated. With the Pt nanoparticles decorated on the surface, the aggregated particles are inefficient to change the inherent surface trap states possibly owing to the deep-level defects, while atomic Pt substitution does not induce more defects in hematite (Supplementary Fig. 25 ). Further on, the high charge transfer efficiency of k trans /( k trans + k rec ) can be obtained on SAs Pt:Fe 2 O 3 , especially in the potential range of 0.8-1.1 V RHE (Fig. 5c ), suggesting that the charge recombination is greatly reduced via single atomic bulk and surface doping. In other words, Pt-O coordination favors the photoresponse at low potentials. Fig. 5: IMPS and TAS for Fe 2 O 3 , NPs Pt/Fe 2 O 3 , and SAs Pt:Fe 2 O 3 . a Charge transfer rate constant ( k trans ); b charge recombination rate constant ( k rec ); c charge transfer efficiencies extracted from IMPS analysis; d , e transient absorption decays observed at d 600 nm and e 700 nm. The fits for the decays were calculated with three exponential decay model, shown as the solid lines, and the circles represent experimental data; f time-resolved transient absorption spectra of SAs Pt:Fe 2 O 3 when excited with 380 nm; g – i electron trapping, electron detrapping, hole trapping, and charge recombination of g Fe 2 O 3 , h NPs Pt/Fe 2 O 3 , and i SAs Pt:Fe 2 O 3 . Full size image TAS can be used to characterize the dynamics of photoinduced charge carrier. The distinct absorption spectra of photoelectrons and holes in photoanode make it possible to monitor the concentration variation of the species, especially the fates of photoholes and photoelectrons on the timescale of picosecond to microseconds. TAS of hematite principally presents two bands, where a bleach band at a probe wavelength of ~600 nm is ascribed to trapping photoelectrons, and an absorption band of ~700 nm corresponds to photoholes [51] , [52] . Under OCP condition (Supplementary Fig. 26 ), the photogenerated charge carrier dynamics can be associated to the bulk electron-hole recombination since the decay dynamics are faster than the timescale of water oxidation on the surface. From the decay dynamics photoinduced absorption (Fig. 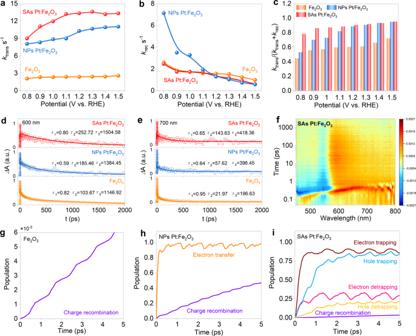Fig. 5: IMPS and TAS for Fe2O3, NPs Pt/Fe2O3, and SAs Pt:Fe2O3. aCharge transfer rate constant (ktrans);bcharge recombination rate constant (krec);ccharge transfer efficiencies extracted from IMPS analysis;d,etransient absorption decays observed atd600 nm ande700 nm. The fits for the decays were calculated with three exponential decay model, shown as the solid lines, and the circles represent experimental data;ftime-resolved transient absorption spectra of SAs Pt:Fe2O3when excited with 380 nm;g–ielectron trapping, electron detrapping, hole trapping, and charge recombination ofgFe2O3,hNPs Pt/Fe2O3, andiSAs Pt:Fe2O3. 5d–f ), the carrier dynamics for the samples was calculated by fitting the kinetics traces at 600 nm and 700 nm (Supplementary Table 5 ). The charge carrier decay average lifetime of τ av at 600 nm extends from 304.49 ps (Fe 2 O 3 ) to 437.28 ps for NPs Pt/Fe 2 O 3 and 486.76 ps for SAs Pt:Fe 2 O 3 . The increased charge carrier decay lifetime of the absorption signal indicates that single atom doping can effectively promote charge separation, extend charge carrier decay lifetime, and reduce the charge recombination on the picosecond time scale. SAs Pt:Fe 2 O 3 shows the long lifetimes at 600 and 700 nm relative to NPs Pt/Fe 2 O 3 and Fe 2 O 3 , indicative of the long-lived photoholes for water oxidation. The pristine Fe 2 O 3 exhibits a fast decay among all samples due to the serious electron-hole recombination. These provide strong evidence that the charge recombination kinetics can be greatly suppressed by SAs Pt doping, which favors to the water photo-oxidation of hematite under the present experimental conditions. We next carried out the nonadiabatic (NA) molecular dynamics with decoherence-induced surface hopping (DISH) approach to analysis the charge carrier dynamics of hematite, and the simulated data are shown in Fig. 5g–i . 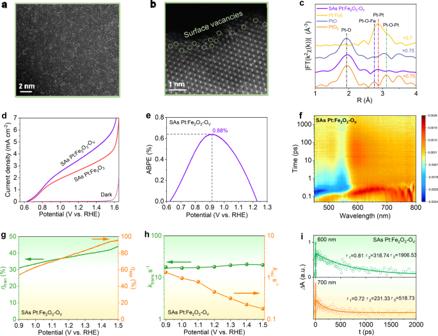Fig. 6: Performance improvement of SAs Pt:Fe2O3-Ov. a,bHigh resolution HAADF STEM images;ck3-weighted Fourier-transform spectra from EXAFS;dJ-Vcurves in 1 M KOH under AM 1.5G illumination;eABPE value;ftime-resolved transient absorption spectra when excited with 380 nm;gcharge separation and charge transfer efficiencies;hcharge transfer rate constants (ktrans)and charge recombination rate constants (krec);itransient absorption decays observed at 600 and 700 nm. The fits for the decays were calculated with three exponential decay model, shown as the solid lines, whereas the circles represent experimental data. Fitting the curves to an exponent, \(P\left(t\right)=\exp (-\frac{t}{\tau })\) , we obtained the charge trapping, detrapping, transfer, and recombination time scales (Supplementary Table 6 ). In general, electron-hole recombination results in short carrier lifetime and reduces OER performance. In the pristine Fe 2 O 3 system, the photogeneration charge carriers occur the detrimental recombination process (Fig. 5g ). Doping the Fe 2 O 3 with Pt NPs (Fig. 5h ), free carrier recombination process is inhibited compared to the Fe 2 O 3 system, and the electron transfer between Fe 2 O 3 and NPs Pt becomes the main process. The fast charge transfer promotes efficient charge separation and prolongs the carrier lifetime. Changing the NPs Pt to SAs Pt (Fig. 5i ), the occurrence of free carrier recombination is further reduced compared to NPs Pt/Fe 2 O 3 system, and the charge carriers mainly take place in trapping and detrapping processes. The charge trapping and detrapping are in dynamic equilibrium, which extends the carrier lifetime and improves the OER performance of Fe 2 O 3 comparable to NPs Pt doping, demonstrating the above experimental results. Further PEC performance enhancement via surface oxygen vacancies Benefited from the role of single atom substitution, we further used plasma etching treatment to produce surface oxygen vacancies (O V ) and accelerate the charge transfer on SAs Pt:Fe 2 O 3 (remarked as SAs Pt:Fe 2 O 3 -O V ). No evident morphology change can be discerned for the treated sample (Supplementary Fig. 27 ). Single atoms are still retained from HAADF-STEM observation (Fig. 6a ). Surface vacancies can be viewed as marked by the circle (Fig. 6b ), accompanied by the irregular surface boundary originated from plasma treatment (Supplementary Fig. 28 ). Moreover, SAs Pt:Fe 2 O 3 -Ov maintains two peaks at 1.96 Å and 2.86 Å in the Pt L -edge EXAFS spectrum (Fig. 6c ), representing the coordination of Pt-O and Pt-O-Fe (Supplementary Fig. 29 ). The slight decrease in peak intensity on SAs Pt:Fe 2 O 3 -O V can be observed compared with SAs Pt:Fe 2 O 3 (Supplementary Fig. 30 ), reflecting a decrease in the coordination number of Pt to O ascribed to the presence of oxygen vacancies. The SAs Pt:Fe 2 O 3 -O V displays Pt-O bonding with CN approaching to 4 at 1.96 Å in the first coordination shell (lower than SAs Pt:Fe 2 O 3 with CN of 4.5), while Pt-O-Fe bonding with CN approaching 1 at 2.86 Å in the second coordination shell (Supplementary Table 7 ). The fitting results of χ ( R ) and χ ( k ) space spectra with reasonable R -factor quantitatively support the local atomic structure and coordination numbers information. O 1s XPS spectrum shows that the lattice oxygen is shifted to higher binding energy by 180 mV for SAs Pt:Fe 2 O 3 -O V , while Pt 4f XPS spectrum is negatively shifted after plasma treatment (Supplementary Fig. 31 ). This means that SAs Pt in Fe 2 O 3 -O V are electron-richer compared with SAs Pt:Fe 2 O 3 , and more charge can be transferred from Fe 2 O 3 to Pt. Additionally, Pt content on the top surface has decreased from 9.96 (without plasma treatment) to 6.97 at.% (Supplementary Table 8 ). This can be originated from the generated surface O V , which anchors the Pt single atom to stabilize it. Fig. 6: Performance improvement of SAs Pt:Fe 2 O 3 -Ov. a , b High resolution HAADF STEM images; c k 3-weighted Fourier-transform spectra from EXAFS; d J-V curves in 1 M KOH under AM 1.5G illumination; e ABPE value; f time-resolved transient absorption spectra when excited with 380 nm; g charge separation and charge transfer efficiencies; h charge transfer rate constants ( k trans )and charge recombination rate constants ( k rec ); i transient absorption decays observed at 600 and 700 nm. The fits for the decays were calculated with three exponential decay model, shown as the solid lines, whereas the circles represent experimental data. Full size image The PEC performance of SAs Pt:Fe 2 O 3 -O V is further improved after optimization (Supplementary Fig. S32 ), in which the photocurrents reach to 3.65 and 5.30 mA cm -2 at 1.23 and 1.5 V RHE with a maximum ABPE value of 0.68% (Fig. 6d, e ). This is more than double the previously reported highest value of the doped Fe 2 O 3 -based photoanodes (Supplementary Table 1 ), and even superior to the cocatalysts decorated Fe 2 O 3 -based photoanodes (Supplementary Table 9 ). Meanwhile, V on shifts to the negative direction with ∆ V on = 5 mV, in line with the negative shift of the flat band potential on SAs Pt:Fe 2 O 3 -O V deduced from the Mott–Schottky plot (Supplementary Fig. 33 ). This is currently known as one of the best performances in terms of photocurrent and V on for elemental doping hematite semiconductors. Moreover, the electrochemical specific surface area of SAs Pt:Fe 2 O 3 -O V is evidently increased, almost 4 times higher than that of the SAs Pt:Fe 2 O 3 (Supplementary Fig. 34 ). There is no notable enhancement on the charge separation between SAs Pt:Fe 2 O 3 -O V and SAs Pt:Fe 2 O 3 , but the charge transfer efficiency of SAs Pt:Fe 2 O 3 -O V highly increases (Fig. 6g and Supplementary Fig. 35 ), supporting the charge transfer influenced by the oxygen vacancies. The charge carrier derived from OCP displays that SAs Pt:Fe 2 O 3 -O V has faster photoresponse (Supplementary Fig. S36 ), along with higher k trans value, lower k rec values (Fig. 6h and Supplementary Fig. 37 ), and long charge carrier lifetime (Fig. 6f, i ) comparable with non-treated SAs Pt:Fe 2 O 3 (Supplementary Fig. 38 ). The surface recombination is generally happened which affects the oxygen evolution reaction and PEC activity of the photoelectrode. Here the surface oxygen vacancies induced can serve as surface states below the conduction band minimum that boost the charge carrier transfer. The defects raise the flat band potential away from the redox potential of O 2 /H 2 O and increase the upward bending of the hematite band edge. This can facilitate the charge transfer from the Fe 2 O 3 surface to the electrolyte. In other words, surface oxygen vacancies are conductive to a reduced interfacial charge-transfer barrier and surface trapping states. PDOS of SAs Pt:Fe 2 O 3 -O V demonstrates that oxygen vacancies can eliminate the trap states between the band gap of Fe 2 O 3 (Supplementary Fig. 39a, b ), reducing the charge recombination. Also, ELF (Supplementary Fig. 39c ) shows that oxygen vacancies noticeably reduce electron localization and electron transport resistance, which act as active sites for chemisorption of the intermediates, and improve the surface water ability. All these results demonstrate that the synergistic effect of single atom coordination and surface oxygen vacancies are responsible for the improved charge transfer and the suppressed photogenerated charge recombination, boosting water oxidation ability. Based on the calculation and experimental results above, a mechanism is proposed to clarify the improved charge carrier kinetics for SAs Pt decorated on the defected Fe 2 O 3 . The influence of charge transfer and recombination is schematically illustrated in Supplementary Fig. 40 . When Fe 2 O 3 is exposed to light to generate photo-generated carriers, most of the photo-generated carriers would be recombined instantaneously before arriving to the surface for water oxidation reaction owing to the short hole diffusion length. Few separated photogenerated electrons and holes in the conduction band and the valence band are transferred to the corresponding surface to participate in oxygen and hydrogen evolution reactions, causing the poor performance. When Pt species were incorporated to Fe 2 O 3 , the mobility of excited carrier can be accelerated, thereby improving the carrier transfer efficiency. In contrast to the traditional element doping, single atoms coordination is in favor of improving the charge separation efficiency and prolonging the charge carrier lifetime by the shift of the photogenerated holes towards the photoanode/electrolyte interface and of the electrons to the back side. On the other hand, single atom-level substitution can efficiently suppress the deep-level defects in hematite relative to the nanoparticle/cluster-level doping, in which the latter with aggregated defects has a distribution along the photoanode. Further surface oxygen vacancies were produced in the material, thereby surface oxygen vacancies and reduced Fe 2+ species within the nanoflakes following the doping reaction mechanism. In addition, one-dimensional single-crystalline nanoflakes structure with enough light harvesting could facilitate the charge collection efficiency. In summary, single platinum atom doped into Fe 2 O 3 photoanode has been successfully synthesized by using 2,2-bipyridine as the ligand to chelate Pt cations, followed by the inert atmosphere treatment. Compared with NPs Pt loading, SAs Pt:Fe 2 O 3 can obviously suppress the deep-level defects and shift the band edge positions of Fe 2 O 3 . The introduction of surface oxygen vacancies further enhances the PEC activity of the SAs Pt:Fe 2 O 3 . The resulting photoanode achieves the photocurrent densities of 3.65 and 5.30 mA cm −2 at 1.23 and 1.5 V RHE with a high ABPE of 0.68% for the hematite-based photoanodes. The synergism of single atomic-level doping and surface oxygen vacancies improve charge carrier separation capability and injection efficiency at the semiconductor/electrolyte interface, prolong the charge carrier lifetime, and promote the reaction kinetics. These results clarify the importance of the designing single atom doping engineering in the photoelectrode to boost the efficient charge transfer and extending charge lifetime, and provide a design idea to construct highly efficient photoelectrodes for improving the solar conversion efficiency of other semiconductors. Material preparation Iron foils (Alfa Aesar, 0.25 mm thick, 99.99%) with a size of 1 cm 2 were degreased by ultrasonic treatment in acetone and ethanol for 10 min, and then dried in a nitrogen stream. To prepare the α-Fe 2 O 3 nanoflakes grown on iron substrate, iron foils were thermally annealed in a furnace (HF-Kejing Furnace, KSL-1100X) at 400 °C in air at a heating rate of 10 °C min −1 and kept at the required temperature for 3~4 h. The entire sample surface became nanoflakes during the thermal annealing for the following treatment. Hexachloroplatinic acid hexahydrate (5 mmol) dissolved in ethanol was mixed with 2,2-bipyridine in a molar ratio of 1:1, 1:3, and 1:6 for 10 min The α-Fe 2 O 3 nanoflakes were immersed into the above solution for different times (5 min, 15 min, 25 min, and 35 min), following by drying overnight in a vacuum oven at 60 °C. Next, the samples were annealing in Ar at 330 °C and 400 °C for 100 min for the synthesis of SAs Pt:Fe 2 O 3 and NPs Pt/Fe 2 O 3 , respectively. For the SAs Pt:Fe 2 O 3 -O V , SAs Pt:Fe 2 O 3 was treated in a plasma etching condition (HF-Kejing, PEC-500 W) in Ar at 20 W for various times (5 min, 15 min, 25 min, and 35 min). Photoelectrochemical characterization Photoelectrochemical measurements were measured in a standard three-electrode system with a CHI 760D electrochemical analyzer. The light source was used the simulated AM 1.5 G (100 mW cm −2 ) sunlight. The solar simulator used for PEC measurement was equipped with a total-reflection mirror and AM 1.5G fitter, and the spectrum was measured as shown in Supplementary Fig. 41 . 1 M Potassium hydroxide (KOH, pH = 14) was used as an electrolyte. The prepared sample, Pt foil, and Ag/AgCl were used as the working electrode, counter electrode, and reference electrode, respectively. Photocurrent vs voltage ( I-V ) curves were recorded by scanning the potential from −0.5 to 0.65 V Ag/AgCl with a rate of 10 mV s −1 . The measured potential was converted into a potential with respect to a reversible hydrogen electrode (RHE). There is no iR correction performed in the experiment. Electrochemical impedance spectroscopy (EIS) was performed at 1.23 V RHE and a small AC amplitude of 10 mV in the frequency range of 10 −2 –10 5 Hz under AM 1.5 G illumination. Applied bias photon-to-current efficiency (ABPE) can be calculated using the following equation of ABPE (%) = \(\frac{J\times \left(1.23-{V}_{b}\right)}{{p}_{{total}}}\) , in which J is the photocurrent density (mA cm −2 ) obtained from AM 1.5G illumination, V b refers to the applied bias potential versus RHE, and P total is the total light intensity of AM 1.5 G. The incident photoelectron conversion efficiency (IPCE) was measured in 1 M KOH at a potential of 1.23 V RHE in a Xe lamp. IPCE was calculated using the formula of IPCE (%) = \(\frac{J\times 1240}{\lambda \times {p}_{{Light}}}\times 100\%\) , where J presents the photocurrent density (mA cm −2 ), λ and P light are the incident light wavelength (nm) and the power density obtained at a specific wavelength (mW cm −2 ), respectively. Charge separation efficiency ( η sep , the yield of photo-generated holes reaching the semiconductor/electrolyte interface) and surface charge transfer efficiency ( η trans , the yield of holes participating in the water oxidation reaction after reaching the electrode/electrolyte interface) can be calculated using the following formula of η sep = \(\frac{{J}_{{H}_{2}O}}{{J}_{H2O2}}\) and η trans = \(\frac{{J}_{H2O2}}{12.5}\) , in which J H2O and J H2O2 are the photocurrent densities obtained in 1 M KOH without and with H 2 O 2 , 12.5 mA cm −2 is the theoretical photocurrent of Fe 2 O 3 under AM 1.5 G illumination. For comparison of charge recombination rate at the photoanode/electrolyte junction, the carrier lifetime was quantified by τ n ( τ n = \(\frac{{K}_{B}}{e}({\frac{{dOCP}}{{dt}}})^{-1}\) ). Material characterization The crystalline structure and composition were performed by X-ray diffraction analysis (XRD, Rigaku RINT-2000, Cu K α radiation at 40 kV and 40 mA) and X-ray photoelectron spectroscopy (XPS, ESCALAB 250xi, Thermo Fisher Scientific). The elemental contents were tested by inductively coupled plasma optical emission spectroscopy (ICP-OES-720ES, Agilent, USA). The morphology was observed using field emission scanning electron microscopy (FE-SEM, Supra 55, Zeiss, Germany) and transmission electron microscopy (TEM, JEM-2100F, JEOL, Japan) systems. The cross-sectional SEM image was taken by argon-ion milling machine (GATAN, ILION693) with a voltage of 5 kV, following with SEM observation. The aberration-corrected high-angle annular dark-field scanning transmission electron microscopy was performed using JEM-ARM200F. UV-visible diffuse reflectance spectra were implemented on a UV-2600 (Shimadzu) spectrometer using BaSO 4 as the reference. Photoluminescence (PL) spectra were performed on a HORIBA Fluoromax-4 (HORIBA JY, HORIBA Fluoromax-4, USA) under laser excitation at 350 nm. The electron paramagnetic resonance (EPR) measurements were recorded using a JES-FA200 spectrometer at low temperature (−150 °C). Charge carrier kinetics measurements Intensity modulated photocurrent spectroscopy (IMPS) was performed with a potentiostat (PGSTAT302N, Metrohm), an impedance analyser (FRA32M, Metrohm), and a light-emitting diode (LED) driver kit (Metrohm) that drove illumination of 420 nm power UV LED in 1 M KOH at different voltages (0.8 V RHE , 0.9 V RHE , 1.0 V RHE , 1.1 V RHE , 1.2 V RHE , 1.3 V RHE , 1.4 V RHE , and 1.5 V RHE ). The LED intensity was 5.5 mW cm −2 , and it was modulated by 10% in the range of 10 kHz–0.1 Hz. Transient absorption spectroscopy (TAS) measurements were performed on a Helios (Ultrafast systems) spectrometers using a regeneratively amplified femtosecond Ti:sapphire laser system (Spitfire Pro-F1KXP, Spectra-Physics; frequency, 1 kHz; max pulse energy, ~8 mJ; pulse width, 120 fs) at room temperature. For the TAS sample preparation of the pristine hematite, ten pieces of Fe 2 O 3 nanoflakes with the same experimental condition were scratched from the iron foils into a 5 ml sample storage using a plastic dropper. Then, 3 ml deionized water was added into the storage, and was ultrasonic treated for 30 min to maintain high dispersion of the sample. For comparison, we conducted the TAS measurement of the deionized water to eliminate its disturbance during the measurement. The TAS sample preparations of NPs Pt/Fe 2 O 3 and SAs Pt:Fe 2 O 3 were used the same treatment of the pristine Fe 2 O 3 . The data were analyzed through commercial software (Surface Xplorer, Ultrafast Systems). An individual three-exponential decay model was used to calculate the fits of the decay. The amplitude weighted average lifetime ( τ av ) can be fitted using the following equation of τ av= \(\frac{{{{{{\rm{SUM}}}}}}[{Ai}\times \tau i{]}}{{{{{{\rm{SUM}}}}}}[{Ai}{]}}\) , where A i is the amplitude of the component with lifetime ( τ i ), and τ i is the amplitude weighted lifetime. Simulation methodology Geometry optimization, electronic structure, adiabatic molecular dynamic (MD), and nonadiabatic (NA) coupling calculations were performed using Vienna ab initio simulation package (VASP) software [53] . The electron exchange-correlation and electron-ion core interactions were treated with the generalized gradient approximation of Perdew–Burke–Ernzerhof (PBE) [54] and projector-augmented-wave (PAW) [55] approaches, respectively. Typically, the Fe 3d strong correlated electrons cannot be well-described by the standard DFT method. Therefore, to correct the strongly correlated electronic nature of Fe 3d-electrons, we applied the on-site Coulomb correction (U = 5 eV for Fe 3d orbitals) to accurately describe the band gap of Fe 2 O 3 (~2.0 eV), which agrees well with the data (2.1 eV) calculated using the same functional method [56] . The plane wave cutoff energy was set to 500 eV. The weak van der Waals interactions were described with the Grimme DFT-D3 methdsh [57] . The geometry optimizations were carried out at Γ-point because a large supercell was used. The electronic structure calculations were performed on 2 × 2 × 1 grid for k-point sampling. After the geometry optimization, all systems were heated to 300 K by repeated velocity scaling. Then, 4 ps microcanonical ensemble adiabatic MD trajectories were obtained. The nonadiabatic molecular dynamic (NAMD) simulations were calculated with the decoherence-induced surface hopping (DISH) method [58] implemented within the time-dependent Kohn–Sham density functional framework [59] , [60] , [61] , which were performed using the PYthon eXtension for Ab Initio Dynamics (PYXAID) code [62] , [63] . The four-electron OER occurs based on Equations (1)–(4), where the * represents the surfaces: 
    ∗+H_2O→*OH+e^-+H^+
 (1) 
    *OH→*O+e^-+H^+
 (2) 
    H_2O+∗O→ *OOH+e^-+H^+
 (3) 
    *OOH→∗+O_2+e^-+H^+
 (4) The Gibbs free energy \(G\) was calculated with the followed equation of \(G=\,E+\,{E}_{{ZPE}}-{TS}-{eU}\) . \(E\) , \({E}_{{ZPE}}\) , \(S,\) \(U,\) and \({T}\) correspond single point energy, zero-point energy, entropy, potential versus standard hydrogen electrode, and temperature (298.15 K), respectively. The overpotential ( η ) toward OER was computed using the equation ( U = 0 V) of η \(=\frac{{{\max }}\left\{\Delta G1,\Delta G2,\Delta G3,\Delta G4\right\}}{e}-1.23.\) The \(\Delta G1,\Delta G2,\Delta G3,\,{{{{{\rm{and}}}}}}\,\Delta G4\) represent the Gibbs free energy difference for elementary reactions.